Self-adaptive strain-relaxation optimization for high-energy lithium storage material through crumpling of graphene High-energy lithium battery materials based on conversion/alloying reactions have tremendous potential applications in new generation energy storage devices. However, these applications are limited by inherent large volume variations and sluggish kinetics. Here we report a self-adaptive strain-relaxed electrode through crumpling of graphene to serve as high-stretchy protective shells on metal framework, to overcome these limitations. The graphene sheets are self-assembled and deeply crumpled into pinecone-like structure through a contraction-strain-driven crumpling method. The as-prepared electrode exhibits high specific capacity (2,165 mAh g −1 ), fast charge-discharge rate (20 A g −1 ) with no capacity fading in 1,000 cycles. This kind of crumpled graphene has self-adaptive behaviour of spontaneous unfolding–folding synchronized with cyclic expansion–contraction volumetric variation of core materials, which can release strain and maintain good electric contact simultaneously. It is expected that such findings will facilitate the applications of crumpled graphene and the self-adaptive materials. High energy- and power-density rechargeable batteries are in high demand for energy storage systems [1] , [2] , [3] , [4] . Commercialized materials of lithium ion batteries, such as graphite, LiCoO 2 and LiFePO 4 , have limited capacity due to their intercalation mechanism. Beyond mechanism limitations, conversion and alloying reaction-based electrode materials usually have higher capacity over 1,000 mAh g −1 , owing to their multiple electrons transfer per redox centre (two to six electron transfer for conversion and alloying reaction versus no more than one electron transfer for intercalation reaction) [1] , [5] , [6] , [7] , [8] . However, particle pulverization that results from the inherent large volume variations ( Fig. 1a and Supplementary Fig. 1 ), combined with intrinsically sluggish charge and mass transfer kinetics, can seriously limit the cycling, rate performance and further applications [5] , [9] , [10] , [11] . To buffer the large volume expansion and enhance their kinetics, much research has focused on conductive encapsulation, mostly through carbon or conductive polymer coating [12] , [13] . However, collapse of the shell and increasing of core-shell interspaces during long cycles will induce structure damage, conductivity deteriorating and further lead to the electrochemical performance fading ( Fig. 1b ). To construct robust protection for large-volume-change materials, our group designed and synthesized semihollow bicontinuous graphene scrolls to protect the nanowire structure and show an enhanced capacity retention [14] . Cui’s group created yolk-shell nanoarchitecture [15] , [16] , pomegranate-inspired structure [17] to provide free-space for large volumetric expansion and impede solid-electrolyte interphase formation. Distinction of our work and previous reports [14] , [15] , [16] , [17] , [18] , [19] is that we propose a further-optimized and novel electrode with more stretchy protective shell and sustainable core-shell contact rather than void space, yielding rapid strain-relaxation and sustainable electric contact simultaneously. 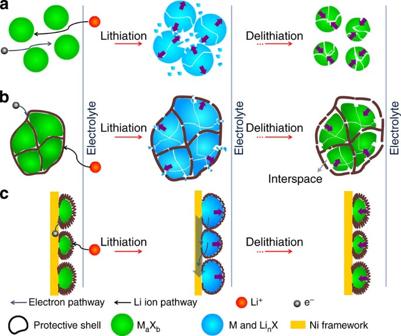Figure 1: Schematics of the electrochemical process in various configuration electrodes. (a) Bare particles undergo large volumetric change and tend to pulverize during cycling, resulting in poor cycling and rate performance. (b) Core–shell morphology provides a protective coating, but cracking of the shell as well as increasing of interspace between core and shell will occur on volume expansion and contraction. (c) In cG-encapsulated 3D bicontinuous electrode, reversible unfolding/folding of cG buffers volume expansion and 3D configuration enhances the transport efficiency, resulting in high cycling stability and rate capability. Figure 1: Schematics of the electrochemical process in various configuration electrodes. ( a ) Bare particles undergo large volumetric change and tend to pulverize during cycling, resulting in poor cycling and rate performance. ( b ) Core–shell morphology provides a protective coating, but cracking of the shell as well as increasing of interspace between core and shell will occur on volume expansion and contraction. ( c ) In cG-encapsulated 3D bicontinuous electrode, reversible unfolding/folding of cG buffers volume expansion and 3D configuration enhances the transport efficiency, resulting in high cycling stability and rate capability. Full size image To realize the sustainable contact of optimized electrode, one of the optimal approaches is the utilization of ‘self-adaptive materials’. To our knowledge, the concept of ‘self-adaptive materials’ was first proposed in 1994: if a two-dimensional elastic continuum for minimum compliance subject to a constraint on the total volume of material, which is termed self-adaptive behaviour, the material can obtain the optimal strain relaxation [20] . However, due to the lack of the ideal materials and/or appropriate synthetic methods, this kind of material or behaviour was seldom reported. On the other side, to realize the stretchy protective shell, crumpled graphene (cG) has been recently demonstrated to possess high stretch ability, more active sites and ultrafast mass transfer [21] , [22] , [23] , [24] , [25] , [26] . These advantages indicate that cG could offer unprecedented opportunities to serve as stretchy shell for conversion or alloying-based electrode materials. To maximize the potential and utilization of cG as protective shell in electrochemical devices, it is crucial to establish an effective synthetic strategy to deeply crumple the graphene shell. Moreover, comprehensive characterization and incisive theoretical analysis, such as in situ and ex situ electron microscopic characterization, theoretical simulation, should be applied to study the new strain-relaxation behaviours in folding–unfolding process. In this work, we describe the design of cG encapsulated three-dimensional (3D) electrode ( Fig. 1c ) through a contraction-strain-driven crumpling method during liquid–solid transition of encapsulated particles. The crumpled construction combined with 3D framework yields significant improvements in the cycling stability and rate performance for Li batteries. Further structural analysis and mechanism studies followed by ex situ scanning electron microscopy (SEM), ex situ and in situ transmission electron microscopy (TEM) and molecular dynamics (MD) simulations, suggest that this strategy can overcome the aforementioned limitations of electrode materials, and more importantly, reveal that cG shells have self-adaptive behaviour, which provides new insights for understanding and applications of cG. Synthesis and characterization of the electrode To achieve the cG-encapsulated 3D bicontinuous framework Ni 3 S 2 electrode (Ni 3 S 2 @cG/Ni, here Ni 3 S 2 is served as a typical conversion reaction material due to their high theoretical capacities, good safety and cost effectiveness [19] ). Our fabrication process involves three overall stages (schematics, Fig. 2a ): (1) Synthesis of graphene oxide encapsulated sulphur particles (S@GO) through the well-controlled reaction of sodium polysulphides with hydrochloric acid. The synthesized sulphur can adhere to and self-assemble on the negatively charged graphene sheets when GO was dispersed in solution. (2) Fabrication of graphene oxide-encapsulated 3D bicontinuous framework electrode by a one-step hydrothermal process using pretreated 3D nickel framework and the as-prepared S@GO nanoparticles. (3) Reducing the GO shell to graphene by hydrazine solution and hydrogen plasma. To better investigate the effect of cG on electrochemical performance, bare Ni 3 S 2 3D electrode (Ni 3 S 2 /Ni, replacing S@GO by sulphur powder and other conditions were the same as synthesis of Ni 3 S 2 @cG/Ni) and cG-encapsulated 3D electrode with half content of graphene (Ni 3 S 2 @0.5 cG/Ni, reducing the graphene to half in the synthesis of graphene encapsulated sulphur and other conditions were same as synthesis of Ni 3 S 2 @cG/Ni) were fabricated as control experiments. 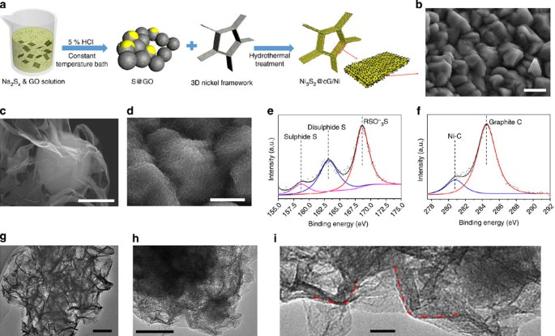Figure 2: Synthesis and characterization of cG-encapsulated 3D Ni3S2electrode (Ni3S2@cG/Ni). (a) Fabrication process of Ni3S2@cG/Ni electrode, including preencapsulating sulphur with graphene oxide and one-step hydrothermal reaction with 3D nickel framework. (b) Low-magnification SEM image of Ni3S2@cG/Ni. (c) SEM image of S@GO. (d) Zoom-in SEM image of Ni3S2@cG/Ni, the cG with sharp ridges encapsulate the micrometre-sized particles. (e,f) XPS of S 2p, C 1s spectra of electrode surface. TEM images of (g) cG shell, (h,i) Ni3S2@cG which derive from the surface of Ni3S2@cG/Ni electrode. High-resolution TEM image (i) showed the bend of crystal lattice (marked with red line) of graphene, which indicates the crumple in graphene. Scale bars (b) 1 μm, (c,d) 500 nm, (g) 200 nm, (h) 50 nm, (i) 10 nm. Figure 2: Synthesis and characterization of cG-encapsulated 3D Ni 3 S 2 electrode (Ni 3 S 2 @cG/Ni). ( a ) Fabrication process of Ni 3 S 2 @cG/Ni electrode, including preencapsulating sulphur with graphene oxide and one-step hydrothermal reaction with 3D nickel framework. ( b ) Low-magnification SEM image of Ni 3 S 2 @cG/Ni. ( c ) SEM image of S@GO. ( d ) Zoom-in SEM image of Ni 3 S 2 @cG/Ni, the cG with sharp ridges encapsulate the micrometre-sized particles. ( e , f ) XPS of S 2p, C 1s spectra of electrode surface. TEM images of ( g ) cG shell, ( h , i ) Ni 3 S 2 @cG which derive from the surface of Ni 3 S 2 @cG/Ni electrode. High-resolution TEM image ( i ) showed the bend of crystal lattice (marked with red line) of graphene, which indicates the crumple in graphene. Scale bars ( b ) 1 μm, ( c , d ) 500 nm, ( g ) 200 nm, ( h ) 50 nm, ( i ) 10 nm. Full size image The GO used in first stage was characterized by Raman spectrum and atomic force microscopy (AFM). The Raman peak at 1,351 and 1,590 cm −1 can be indexed to the D and G vibrational bands of graphene ( Supplementary Fig. 2 ). The thickness of GO is determined by AFM is ~1 nm and the width is up to a micrometre ( Supplementary Fig. 3 ). Then, S@GO was characterized by SEM, X-ray diffraction (XRD) and energy diffraction spectroscopy (EDS). The SEM images ( Fig. 2c and Supplementary Fig. 4b,c ) shows that sulphur particles of ~500 nm are randomly covered by GO shells. The main phase detected in XRD of S@GO is sulphur with no obvious diffraction peak of GO ( Supplementary Fig. 4a ). The EDS mappings ( Supplementary Fig. 4e,f ) confirm the presence of sulphur as core and GO as shell. After hydrothermal and reduction process, Ni 3 S 2 @cG/Ni electrode was obtained and characterized by XRD, EDS, SEM, TEM and X-ray photoelectron spectroscopy (XPS). The XRD patterns of Ni 3 S 2 @cG/Ni shown in Supplementary Fig. 5a can be indexed to Ni 3 S 2 (mainphase, JCPDS-ICDD Card No. 00-044-1418), with small amounts of NiS (JCPDS-ICDD Card No. 00-001-1286, marked with ▪) and Ni (JCPDS-ICDD Card No. 03-065-2865, marked with ▴ ). As SEM images shown in Fig. 2b,d , the as-prepared particles with size of ~500 nm are encapsulated by deeply cG layers and compactly stacked on the nickel framework. Compared with the randomly covered S@GO ( Fig. 2c ), graphene in Ni 3 S 2 @cG/Ni is deeply crumpled into a pinecone-like structure, which has a pattern of ridges with wavelength of ~30 nm. TEM and high-resolution TEM images ( Fig. 2g–i and Supplementary Fig. 6 ) captured from cG encapsulated nickel sulphides (Ni 3 S 2 @cG and Ni 3 S 2 @0.5cG) confirm the crumpled nature of graphene. In particular, it is clearly observed that graphene on the boundary of Ni 3 S 2 @cG particles was highly crumpled ( Fig. 2g,h and Supplementary Fig. 6a,b ) and the bent crystal lattice of multi-layered graphene ( Fig. 2i ) was also detected under the high-resolution TEM, which demonstrates the deeply cG encapsulated structure. In contrast, the crumpling degree of graphene in Ni 3 S 2 @0.5 cG is relatively low ( Supplementary Fig. 6c,d ) and even some non-cG or bare particles can be observed ( Supplementary Fig. 6g ). The chemical bonding interaction among Ni 3 S 2 , cG and nickel framework is characterized by XPS ( Fig. 2e,f ). The S 2p ( Fig. 2e ) peaks can be resolved into three components centered at about 157.8, 162.8 and 167.8 eV and represent sulphide, disulphide and RSO 3 − S group, corresponding to the NiS, Ni 3 S 2 and cG, respectively. Similarly, the bonding signals of Ni-C, graphite C can be detected from the C 1s spectrum ( Fig. 2f ). In particular, the RSO 3 − S, Ni-C signals can be assigned to the chemical bonding of cG-Ni 3 S 2 and cG-Ni, which can improve the interfacial stability. Crumpling mechanism The cG has been realized in previous studies and is thought to be driven by thermal expansion, capillary compression and pre-strain relaxation [27] , [28] , [29] , [30] . In particular, Huang’s group first demonstrated that capillary compression effectively cG into a ball-like structure in rapidly evaporating aerosol droplets process [30] . Distinguished from previous results, the deeply cG-encapsulated materials is synthesized in wet chemistry environment in our experiment that has not been reported previously. Therefore, the chemical bonding interaction and self-assembly need to be taken into full consideration. Here, we carried out TEM characterization on the samples at different reaction stages and MD simulation to demonstrate the crumpling mechanism of graphene. The TEM images of samples with different reaction time ( Supplementary Fig. 7a–h ) show the morphological evolution of Ni 3 S 2 @cG during the synthetic process, which indicates that crumpling degree is increasing with an extension of reaction time. Furthermore, a detailed crumpling process of graphene ( Supplementary Fig. 7i–l, Movie 1 ) is revealed by MD simulation through considering the volume variation and chemical binding interaction between graphene and nanoparticle, which well conforms to the TEM observation (More detailed discussion is provided in Supplementary Information ). As shown in Supplementary Fig. 8 , in the formation process of cG-encapsulated 3D framework electrode, the encapsulated solid sulphur (melting point: 115 °C) firstly melts to liquid state at 180 °C, further covering the GO inner surface by capillary force. Because of the high surface energy-induced thermodynamics instability, GO with encapsulated liquid sulphur tend to adhere to the surface of nickel framework. At the early stage of reaction between liquid sulphur and nickel, solid nickel sulphides (melting point: 797 °C) is formed accompanied with volume contraction. With the phase contact line of liquid and solid receding during volume contraction, the slight crumple firstly emerges and assembles that is driven by adhesion and friction forces between nickel sulphides and graphene layers [31] . Meanwhile, the reaction of nickel sulphides and GO takes place that can be confirmed by the above XPS results. The chemical bonding forces will induce more deep crumpling assembly, because they robustly anchor nickel sulphides particles to the GO and restrain the slide of GO at further volume contraction process. Electrochemical properties To evaluate the electrochemical performance and explore the influence of cG, lithium batteries were fabricated based on the Ni 3 S 2 @cG/Ni, Ni 3 S 2 @0.05 cG/Ni and Ni 3 S 2 /Ni electrodes. The cycling performance of Ni 3 S 2 @cG/Ni electrode was firstly tested at a lower current density of 0.1 A g −1 and 0.5 A g −1 from 1.0 V to 3.0 V for 100 charge/discharge cycles ( Fig. 3a ). This voltage window is selected similar to Li 4 Ti 5 O 12 for good safety [4] , [19] . An initial capacity of 1,036 mAh g −1 can be obtained and stabilized to over 900 mAh g −1 after 100 cycles at a current density of 0.1 A g −1 , which is over five times improvement compared with the commercialized graphite (~200 mAh g −1 ) (ref. 2 ) and Li 4 Ti 5 O 12 (~170 mAh g −1 ) (ref. 32 ). When the current density increases to 0.5 Ag −1 , the specific capacity can reach 682 mAh g −1 and maintain 654 mAh g −1 after 100 cycles, with capacity retention up to 96%, which shows over one order of magnitude improvement compared with Ni 3 S 2 /Ni electrode (~7% capacity retention at 0.5 A g −1 after 100 cycles). The additional reversible capacity beyond their theoretical capacity is mainly contributed by interspatial lithium storage of cG and conversion reaction materials [8] . Crumpling of graphene and newly formed interfaces of metal and lithium sulphides both enlarge the interspatial area and lead to additional capacity. 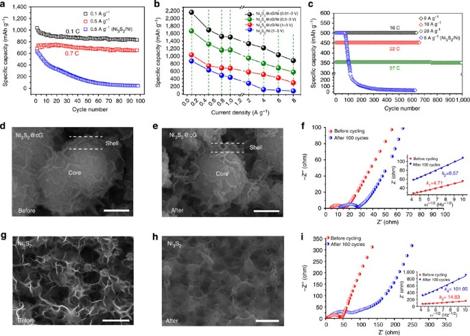Figure 3: Electrochemical performance and morphology characterization before and after charge/discharge cycling. (a) Cycling performance at current density of 0.1, 0.5 A g−1, (b) Rate performance of Ni3S2@cG/Ni and Ni3S2/Ni electrode. (c) Cycling performance at current densities of 8, 10 and 20 A g−1with voltage from 0.01 to 3 V. (d,e) SEM images of Ni3S2@cG/Ni electrode before cycling and after 100 cycles, respectively. (f) Nyquist diagram of Ni3S2@cG/Ni before cycling and after 100 cycles. (g,h) SEM images of Ni3S2/Ni electrode before cycling and after 100 cycles. (i) Nyquist diagram of Ni3S2/Ni before cycling and after 100 charge–discharge cycles. Insets ine,hare the kinetics calculations of Ni3S2@cG/Ni (e), Ni3S2/Ni (h) based on the frequency (ω) andZ' values at low frequency region. Scale bars (d,e,g,h), 500 nm. Figure 3: Electrochemical performance and morphology characterization before and after charge/discharge cycling. ( a ) Cycling performance at current density of 0.1, 0.5 A g −1 , ( b ) Rate performance of Ni 3 S 2 @cG/Ni and Ni 3 S 2 /Ni electrode. ( c ) Cycling performance at current densities of 8, 10 and 20 A g −1 with voltage from 0.01 to 3 V. ( d , e ) SEM images of Ni 3 S 2 @cG/Ni electrode before cycling and after 100 cycles, respectively. ( f ) Nyquist diagram of Ni 3 S 2 @cG/Ni before cycling and after 100 cycles. ( g , h ) SEM images of Ni 3 S 2 /Ni electrode before cycling and after 100 cycles. ( i ) Nyquist diagram of Ni 3 S 2 /Ni before cycling and after 100 charge–discharge cycles. Insets in e , h are the kinetics calculations of Ni 3 S 2 @cG/Ni ( e ), Ni 3 S 2 /Ni ( h ) based on the frequency ( ω ) and Z ' values at low frequency region. Scale bars ( d , e , g , h ), 500 nm. Full size image A summary of the rate performance ( Fig. 3b and Supplementary Figs 9–11 ) with various voltage windows further shows a superb rate capability, and even at higher rate, the Ni 3 S 2 @cG/Ni electrode has larger capacity than Ni 3 S 2 /Ni. In particular, the capacity of Ni 3 S 2 @cG/Ni can reach 2,165 mAh g −1 at a current density of 0.1 A g −1 and 884 mAh g −1 at a current density of 8 A g −1 with voltage from 0.01 to 3.0 V. Additional studies carried out at rates of 8, 10 and 20 A g −1 for extended number of charge–discharge cycles ( Fig. 3c ) yield no capacity fading in 640, 660 and 1,000 cycles, which highlight the substantial improvement afforded by cG compared with baseline Ni 3 S 2 /Ni electrode. In particular, at current density of 20 A g −1 , the power density can reach 18.4 kW kg −1 , five to ten times higher than typical high-power density storage device—supercapacitor [33] . To our knowledge, this maybe one of the best performances among conversion reaction batteries. On the contrary, the Ni 3 S 2 @0.5 cG/Ni and Ni 3 S 2 /Ni electrodes had lower capacity, poorer cycling stability and rate performance ( Fig. 3a,c and Supplementary Figs 9–11 ) due to the lack of sufficient protection from cG. The charge–discharge curves are shown in Supplementary Fig. 9a . The voltage hysteresis, as another important indicator for conversion reaction materials, calculated from the different value between charge and discharge voltage at the half reversible capacity, noted as ΔV(Q/2) , is also investigated and we find that the hysteresis of Ni 3 S 2 @cG/Ni (0.3 V) is much lower than that of Ni 3 S 2 /Ni (0.6 V) at the current density of 0.5 A g −1 . In addition, the ex situ SEM and electrochemical impedance spectrum (EIS) characterizations of Ni 3 S 2 @cG/Ni and Ni 3 S 2 /Ni electrode before and after cycling were carried out to evaluate the structural stability and the kinetics performance of charge and mass transfer. As shown in Fig. 3d , for Ni 3 S 2 @cG/Ni electrode before cycling, the nickel sulphide cores are encapsulated with cG shells. After 100 charge–discharge cycles, although the crumpled GO shells tend to be a bit disordered, the morphology of nickel sulphide core is maintained very well ( Fig. 3e ). As Nyquist diagram shown in Fig. 3f , a low-charge transfer resistance ( R ct ) value can be obtained for Ni 3 S 2 @cG/Ni before cycling, which is reflected by a small diameter of semicircles at the high–medium frequency region. After 100 cycles, the R ct value shows no obvious variation. To assess the lithium ion diffusion kinetics, the calculation based on the impedance data in low frequency region is carried out. According to Supplementary equations (1,2) , the slope in fitting line of ω −1/2 ( ω is frequency) and Z' can be defined as Warburg factor and its square values have an inverse relationship with lithium ion diffusion coefficient ( D Li ). The slope value is 4.72 ( k 1 ) at pristine state and increases to 8.57 ( k 2 ) after 100 cycles, which indicates that D Li degrades to one-fourth of the pristine value. In contrast, for Ni 3 S 2 /Ni electrode, the nickel sulphides are free-standing nanoflakes before cycling ( Fig. 3g ), while serious destruction and significant morphological changes of these nanoflakes occur after 100 cycles ( Fig. 3h ). As Nyquist diagram shown in Fig. 3i , high initial value and large expansion after 100 cycles of R ct can be observed in Ni 3 S 2 /Ni electrode. For the D Li calculation, the Ni 3 S 2 /Ni electrode has a slope value of 14.83 ( k 3 ) before cycling, which indicates that the D Li of Ni 3 S 2 /Ni is an order of magnitude lower than that of Ni 3 S 2 @cG/Ni ( Supplementary equation (1) ). While after 100 cycles, the slope value is 101.05 ( k 4 ) and suggests that D Li degraded to one-fiftieth of the pristine value. According to the above results, we attribute the optimized cycling stability and rate capability to the enhanced transport kinetics and structural stability. First, transport kinetics can be improved through enhancing the electronic conductivity and ionic diffusion efficiency. For the electronic conductivity, the low and relatively stable R ct of Ni 3 S 2 @cG/Ni electrode indicates that 3D conductive framework can sustainably provide continuous ‘highway’ for electron transfer from current collector to active materials. TEM characterization ( Fig. 2g–i and Supplementary Fig. 6 ) of active materials indicates that the cG can construct linkages of electron conduction for separated nickel sulphides particles, so further enhance the electron transfer. For the ionic diffusion, the calculated D Li based on EIS results shows that the Ni 3 S 2 @cG/Ni has about one order of magnitude improvement compared with Ni 3 S 2 /Ni. According to previous reports [34] , [35] , [36] , this improvement is due to the fact that the crumpled structure with enhanced wettability, anisotropic adhesion can realize efficient mass transfer and further yield optimized electric double layer structure. Second, according to the SEM images before and after cycling, the morphology and structure of active materials can be well protected because the deeply cG shell can rapidly relax strain in folding–unfolding process. To further confirm the stabilizing effect and self-adaptive behaviour of the cG shell, we performed ex situ TEM and SEM and in situ TEM characterizations. The batteries were charged/discharged to different voltage states ( Supplementary Fig. 12a ) followed by sampling and ex situ microscopic characterization. As the ex situ TEM ( Fig. 3a,b ) and SEM ( Supplementary Fig. 12b–g ) images showed, the deeply cG spontaneously unfolds and refolds synchronized with the expansion–contraction volumetric variation of core materials. The graphene is highly crumpled at pristine state, then slightly unfolding when discharged to 1.5 V, followed by stretching to a laminated (discharging to 1.0 V) and non-folding (discharging to 0.01 V) shell to adapt the volumetric expansion, which can also refold to deeply crumpled state in recharging process. These results demonstrate that cG has self-adaptive strain-relaxation behaviour by reversible unfolding–folding of crumple. The in situ TEM was performed by constructing an all-solid nanobattery with an active material working electrode, a naturally grown Li 2 O solid electrolyte and a bulk lithium metal counter electrode in TEM chamber ( Supplementary Fig. 13 ). The lithiation is driven by a galvanostat. The lithiation process started when Li 2 O/Li probe contacted with working electrode at 40 s ( Fig. 4d ) and finished at 380 s ( Fig. 4f ). As the lithiation proceeds, the volume continuously expands. And after lithiation, the volume expansion can reach ~170% versus initial state and no pulverization of active materials is observed throughout this process ( Fig. 4c–f , Supplementary Movie 2 ), which can be attributed to the self-adaptive strain relaxation of cG. 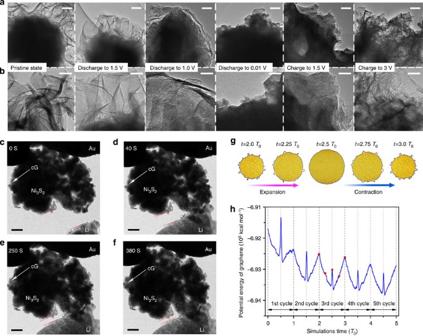Figure 4:Ex situandIn situTEM characterizations and MD simulations of the cG encapsulated electrode. (a) Low magnification and (b) zoom-inex situTEM images of Ni3S2@cG/Ni at different charge/discharge states. Thein situTEM snapshots at (c) 0 s, (d) 40 s, (e) 250 s, (f) 380 s. The distance between the two parallel lines indicates the volume expansion during lithiation process (Details are shown inSupplementary Movie 2). (g) MD snapshots of the graphene encapsulated nanoparticle in the third expansion and contraction cycle. Here, the period of each expansion and contraction cycle isT0. (h) The calculated potential energy of the graphene sheet in a period of five cycles of expansion and contraction. The five red points are corresponding to the five MD snapshots ine(Details are shown inSupplementary Movie 3). Scale bars, (a) 100 nm, (b) 50 nm, (c–f) 200 nm. Figure 4: Ex situ and In situ TEM characterizations and MD simulations of the cG encapsulated electrode. ( a ) Low magnification and ( b ) zoom-in ex situ TEM images of Ni 3 S 2 @cG/Ni at different charge/discharge states. The in situ TEM snapshots at ( c ) 0 s, ( d ) 40 s, ( e ) 250 s, ( f ) 380 s. The distance between the two parallel lines indicates the volume expansion during lithiation process (Details are shown in Supplementary Movie 2 ). ( g ) MD snapshots of the graphene encapsulated nanoparticle in the third expansion and contraction cycle. Here, the period of each expansion and contraction cycle is T 0 . ( h ) The calculated potential energy of the graphene sheet in a period of five cycles of expansion and contraction. The five red points are corresponding to the five MD snapshots in e (Details are shown in Supplementary Movie 3 ). Scale bars, ( a ) 100 nm, ( b ) 50 nm, ( c – f ) 200 nm. Full size image Last, to further understand the stabilizing effect and self-adaptive behaviour of the cG in theory, we carried out MD simulations to investigate the folding–unfolding process of cG with a nanoparticle encapsulated ( Fig. 4g,h and Supplementary Movie 3 ). As shown in Fig. 4h , we plotted the potential energy of the graphene sheet in a period of five cycles of expansion and contraction. This potential energy consists of three parts: the out-of-plane bending energy, the in-plane strain energy and the graphene–nanoparticle interaction energy. According to our simulation results, the last one is fairly small compared with the preceding two terms. In the expansion/contraction process, the cG spontaneously unfolds/folds, which leads to a decrease/increase of the out-of-plane bending energy. We also notice that there is a significant increase of the potential energy at the transition from expansion to contraction. It can be attributed to the fact that ‘tightening hoop effect’ of the enwrapped graphene. As the nanoparticle volume expands, the graphene sheets become suddenly tightened and thus the in-plane strain energy plays a dominant role in the potential energy of graphene sheets. In fact, this increase of the in-plane strain energy is the key to the stabilizing effect of the cG encapsulated 3D electrode. The cG shell could store the strain energy due to the volume expansion during lithiation and release this energy after delithiation. This mechanism is similar to the strength improvement of silicon nanowires encapsulated by a carbon nanotube [37] . But distinguishably, because of the folding–unfolding process, the cG shells can buffer much larger volume variations without structure destruction, and provide sustainable contact between core and shell during the volume expansion–contraction process, which can significantly increase the buffer capacity and enhance the charge/mass transfer kinetics. Making a general survey of the five cycles, it can be seen that the reversible unfolding–folding of cG decreases its potential energy, which indicates a more stable energetic state. We think that the most significant determinant of the stabilizing effect and the self-adaptive behaviour comes from the degree in which graphene sheet wrapped around the nanoparticle. In this sense, the ratio between the circumference of the graphene sheet and the circumference of the nanoparticle, β , is very important. To take into account this effect, we carried out additional MD simulations for various β . ( Supplementary Fig. 14 ). As β decreases, which means the graphene sheet is more tightened, we can find higher potential energy peak at the transition from expansion to contraction, indicating that more strain energy could be stored in the folding–unfolding process. Combining the above characterization and analysis, we can conclude that the cG can spontaneously unfold–fold synchronize with cyclic expansion–contraction volumetric variation of core materials, which can self-adaptively release strain, buffer the electrode volume variations, enhance the structure stability and maintain good electric contact simultaneously. This kind of behaviour cohere well with the concept of ‘self-adaptive behaviour’. Thus, we can attribute this cG to the ‘self-adaptive materials’. In summary, we have demonstrated a robust approach for fabricating and deeply cG-encapsulated 3D electrodes through contraction-strain-driven crumpling during liquid–solid transition of encapsulated particles. The electrode has been tested in lithium batteries. Compared with the electrode without cG encapsulation, this optimized electrode yields significant improvements, especially in the cycling stability and rate capability. This enhanced performance is attributed to the 3D framework providing high continuous electron pathway and more free space for charge and mass transfer, and the stabilizing effect of the cG based stretchy shell. Ex situ and in situ TEM and MD simulations further reveal that the spontaneously unfolding and folding of cG shell can self-adaptively release strain, stabilize the structure during lithiation and delithiation. Those advantages indicate that the optimized electrodes are promising materials to achieve high energy, high-power density and good safety for advanced lithium battery. And more importantly, this deeply cG could offer opportunities to sever as stretchy shell for conversion or alloying-based electrode materials or even used in other fields, such as material protection, bionic design and drug delivery. It is expected that such findings and strategy will facilitate the applications of cG as well as the self-adaptive materials in the future. Materials synthesis Graphene oxide (GO) was synthesized by a modified Hummers method. The concentration of the GO suspension obtained was ~4.7 mg ml −1 , which was determined by drying the suspension at 80 °C under vacuum for 48 h and then weighing the dried GO. Details are described in Supplementary Notes . The GO-coated sulphur particles (S@GO) were synthesized in a facile solution environment through the two-step reaction as follows: Na 2 S+ x S→Na 2 S x +1 , Na 2 S x +1 +2HCl→2NaCl+ x S↓+H 2 S. First, 0.25 g sulphur and 0.65 g Na 2 S·9 H 2 O were added to 50 ml 10 wt.% NaOH solution. The mixture was stirred at 60 °C for 1 h followed by adding 15 ml of graphene oxide (GO) solution. After stirring for 1 h, 5 wt. % HCl was added to adjust pH value to 2 and the precipitation of S@GO was obtained and the products was collected by filtration and dried for 24 h. To investigate the effect of the graphene content on the crumpling morphology and electrochemical performance, the GO-coated sulphur with half-quantity GO (S@0.5GO) was synthesized by adding 7.5 ml GO solution. 3D Ni 3 S 2 @cG/Ni was synthesized by hydrothermal method with S@GO powder and nickel framework followed by reduction of GO shells. The nickel sulphide was formed on the surface of nickel framework substrate by the reaction between nickel and sulphur during hydrothermal process. In detail, a piece of nickel foam disc with a diameter of about 1.8 cm was pretreated by sonicating in ethanol followed by immersing in 2 M HCl for 15 min to get a cleaner and positively charged surface. Then, the pretreated nickel foam disc, 40 mg of S@GO powder and 40 ml of deionized water was transferred to a 100-ml Teflon-lined autoclave at 180 °C for 4 h followed by reducing of GO to graphene with ~0.048 wt.% hydrazine solution (57 μl, 85 wt.% hydrazine dissolved in 100 ml deionized water) and hydrogen plasma treatment. As control experiments, the Ni 3 S 2 @0.5 cG/Ni and Ni 3 S 2 /Ni electrodes were synthesized by adding 40 mg S@0.5GO and 30 mg sulphur powder, while other conditions were same as the synthetic process of 3D Ni 3 S 2 @cG/Ni electrode. Material characterizations The crystal phase of products was characterized by powder XRD. XRD patterns of the products were recorded by a Rigaku D/MAX-III diffractometer with monochromatized Cu K α radiation ( λ =1.5406 Å). The Raman spectrum of GO was taken by confocal Raman microscopy (WITec CRM-200). Field-emission scanning electron microscopy images were collected by a JEOL JSM-7100 F to characterize the morphology of the synthesized nanomaterials. Energy dispersive X-ray mapping was performed on a JEM 2100 F STEM/EDS. Transmission electron microscopic (TEM) images were recorded by a JEOL JEM-2010 microscope at an acceleration voltage of 200 kV. XPS was recorded on VG Multilab 2000. The mass of nickel sulphide and cG on each electrode were determined by testing sulphur and carbon content on Vario EL Cube elemental analyzer. The AFM images was collected using Bruker MultiMode 8 Atomic Force Microscope. Battery assembly and testing Coin cells (2,025) were fabricated in a glove box filled with pure argon gas. Ni 3 S 2 @cG/Ni, Ni 3 S 2 @0.5cG/Ni, Ni 3 S 2 /Ni electrodes directly acted as electrode of coin cells. Specific capacity values were calculated based on the mass of nickel sulphide and cG. The mass of active materials (nickel sulphides and cG) were ~2.0 mg on each electrode, and 5 wt.% of that is graphene ( Supplementary Table 1 ). The capacity contributed from nickel foam substrate can be neglected. Lithium pallet was used as the counter electrode, 1 M solution of LiTFSI in 1,3-dioxolane/Dimethyl Ether (1:1, by volume) was used as the electrolyte. Galvanostatic charge/discharge experiments were performed at several different rates in the potential range of 0.01–3, 0.5–3 and 1–3 V versus Li/Li + with a multichannel battery testing system (LAND CT 2001 A). The long cycling test at current densities of 8, 10 and 20 A g −1 was carried out from 0.01 to 3 V versus Li/Li + with limited capacity of 500, 450 and 350 mAh g −1 , respectively. EIS were carried out with an Autolab electrochemical workstation. The Nyquist diagrams were recorded at batteries’ open potential with frequency range from 0.01 Hz to 100,000 Hz. Ex situ SEM, TEM and in situ TEM The ex situ SEM characterization of electrode before cycling and after 100 times cycling from the disassembled batteries was carried out with the JEOL-7100 F microscope based on the same electrode. The ex situ SEM characterization at different voltage states was performed by charging/discharging a same battery to certain voltages and collecting SEM images on JEOL JSM-7100 F microscope. The ex situ TEM images at different electrochemical states were collected on JEOL JEM-2010 microscope by charging/discharging a same battery to certain voltages. For the in situ TEM characterization, a nanobattery with metallic lithium counter electrode, lithium oxide electrolyte and Ni 3 S 2 @cG nanoparticle working electrode has been constructed inside a JEOL 2010 F TEM using a homemade specimen holder with a nano-manipulator. Individual nanoparticle was attached to a gold wire with a graphite paste. Metallic lithium as the counter electrode was scratched by an electrochemically etched tungsten tip. The oxide layer on the surface of metallic lithium served as the solid electrolyte. Once the Li 2 O-covered Li electrode driven by a nano-manipulator contacted the Ni 3 S 2 @cG nanoparticle electrode, galvanostatic holds of 500 pA were applied across the two electrodes, with respect to the particles lithiation. MD simulations MD simulations were implemented using LAMMPS [38] to explore the fast unfolding of the cG. Our basic modelling setup consisted of a nanoparticle encapsulated by eight pieces of graphene sheets. Here, we choose eight pieces of graphene sheets owing to the compromise with the complicated modelling. It should be noted that there must be some discontinuities in the cG sheet if less or smaller graphene sheets covered on the nanoparticles. A cylindrical model with a diameter of 40 nm was constructed for the nanoparticle. This particular cylindrical model would make it easy to analyse the deformation and reduce the computational time efficiently. Graphene was modelled using the adaptive intermolecular reactive empirical bond order potential [39] . The interactions between carbon atoms and nanoparticles were described by the Lennard–Jones (LJ) potential and the LJ parameters were simply set to be ε =1 meV and σ =3 Å, respectively. The LJ parameter choice is in the appropriate range for typical materials and does not affect the results qualitatively. Since the chemical bonding of cG-Ni 3 S 2 and cG-Ni can be confirmed by the XPS characterization, 5% of the graphene–nanoparticle interactions were enhanced to improve the interfacial stability. The system was equilibrated at 300 K for 0.5 ns using the Nose–Hoover thermostat. After a certain period of time, the graphene sheets wrapped the nanoparticles and the graphene-encapsulated nanoparticle structure can be obtained, as shown in Fig. 4h . From a microscopic perspective, volume variation during charge–discharge cycles implies that the distance between any two atoms in nanoparticles increases and decreases in this process. In our simulations, expansion and contraction processes were simulated by varying the values of LJ parameter σ continuously. The period of each expansion and contraction cycle is T 0 =0.4 ns. All the simulations were performed in the NVT (constant number of atoms, volume and temperature) ensemble. The equations of motion were integrated using a velocity-Verlet scheme with a time step of 2 fs. The snapshots obtained in these simulations were further processed by Atomeye [40] . How to cite this article : Zhao, Y. et al. Self-adaptive strain-relaxation optimization for high-energy lithium storage material through crumpling of graphene. Nat. Commun. 5:4565 doi: 10.1038/ncomms5565 (2014).